Renewable and metal-free carbon nanofibre catalysts for carbon dioxide reduction The development of an efficient catalyst system for the electrochemical reduction of carbon dioxide into energy-rich products is a major research topic. Here we report the catalytic ability of polyacrylonitrile-based heteroatomic carbon nanofibres for carbon dioxide reduction into carbon monoxide, via a metal-free, renewable and cost-effective route. The carbon nanofibre catalyst exhibits negligible overpotential (0.17 V) for carbon dioxide reduction and more than an order of magnitude higher current density compared with the silver catalyst under similar experimental conditions. The carbon dioxide reduction ability of carbon nanofibres is attributed to the reduced carbons rather than to electronegative nitrogen atoms. The superior performance is credited to the nanofibrillar structure and high binding energy of key intermediates to the carbon nanofibre surfaces. The finding may lead to a new generation of metal-free and non-precious catalysts with much greater efficiency than the existing noble metal catalysts. A recent report on the future of carbon dioxide (CO 2 ) emission [1] predicts that in the coming few decades (2010–2060), ~496 gigatonnes of CO 2 will be produced because of fossil fuel combustion by existing infrastructure. Interestingly, CO 2 can be artificially converted into fuel or commodity chemicals [2] , [3] . The CO 2 conversion methodology not only addresses the potential solution for controlling the CO 2 concentration level in the environment but also offers an alternative approach for conversion of renewable energy to a chemical fuel or product. Thus, more research efforts are emphasized towards the CO 2 conversion by electrochemical reduction [4] , [5] , [6] , [7] , [8] , [9] , [10] . So far, various noble metals (Ag [4] , [10] , Au [6] , Cu [7] , Pt [8] and so on) and metal complexes [9] are used as heterogeneous catalysts (as electrodes) for CO 2 reduction. However, the rising cost of noble metals is the main hindrance towards their large-scale practical applications. As a substitute, non-metallic homogenous catalysts (that is, in liquid media) have been significantly studied for the CO 2 reduction [2] , [11] , [12] , [13] . Nevertheless, stability, tedious product separation processes and recovery of the catalyst in these systems still remain among the most problematic issues [14] . On the other hand, a relatively new class of heteroatomic, metal-free heterogeneous catalysts (for example, nitrogen-doped carbon nanotube [15] ) have shown high catalytic performance comparable to noble metal catalysts (for example, platinum) for oxygen reduction reaction (ORR) [15] , [16] , [17] , [18] , [19] . The insertion of heteroatoms (for example, nitrogen and sulphur) [17] in the carbon lattice converts the neutral carbon atoms into positively charged atoms (active sites). It has been claimed that the O–O bond is effectively weakened because of parallel diatomic adsorption of oxygen molecules on these active sites, which promotes the ORR [15] , [16] , [17] , [18] , [19] . However, CO 2 reductions’ mechanistic path is entirely different from the ORR as CO 2 reduction occurs via the formation of intermediate CO 2 complex species, in particular when ionic liquid is used as the electrolyte [4] . Unexpectedly, there are rarely reports on non-metallic heterogeneous catalysts for CO 2 reduction; none have succeeded in demonstrating satisfactory CO 2 reduction ability. In addition, CO 2 reduction mechanism for carbon nitrogen heteroatomic catalysts has not been addressed [20] . In this study, we use low-priced and metal-free carbon nanofibres (CNFs) catalyst synthesized by pyrolysis of electrospun nanofibre mats of heteroatomic polyacrylonitrile (PAN) polymer [21] for CO 2 reduction. The heteroatomic configuration of this catalyst is designed to exploit existing nitrogen atoms in the backbone of precursor (PAN). 1-ethyl-3-methylimidazolium tetrafluoroborate (EMIM-BF 4 ) is chosen as the electrolyte because of its high CO 2 capture ability [22] and CO 2 reduction overpotential-dropping feature [4] . Our non-metallic catalyst system demonstrates the highest performance for CO 2 reduction at low overpotential compared with existing noble metal catalysts to date (for example, ~13 times higher CO 2 reduction current density compared with bulk Ag catalyst). CNFs characterization The CNFs were synthesized by carbonization of electrospun PAN nanofibre mats in argon (Ar) media (see Methods). Macroscopic image of an as-prepared CNFs mat (a defined small piece) is shown in Fig. 1a . The scanning electron microscopic (SEM) image shows the morphological view (at micro scale) of the sample displaying randomly oriented nanofibres in the mat ( Fig. 1b ). The magnified SEM and atomic force microscopic images ( Fig. 1c–e ) deliver more detailed information about the dimensions of the individual fibre (the cross-sectional diameter ~500 nm). The surface roughness along the axis of an individual fibre was also measured resulting in an average surface corrugation with a height of ~15 nm ( Fig. 1f ). The nanocorrugated fractal-like configuration also dramatically increases the effective surface area. High-resolution transmission electron microscopy verified the short-range ordered crystal below few nanometres, which clearly manifests the turbostratic nature of the CNFs [21] . The diffused ring in the selected area electron diffraction pattern (inset in Fig. 1g ) is also consistent with the TEM analysis, confirming the disordered crystal (graphitic) structure of CNFs surface. 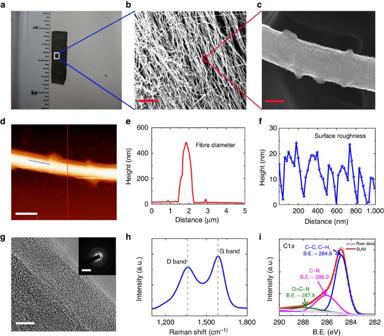Figure 1: Structural and elemental analysis of CNFs. (a) Digital image of CNF mat used as catalyst, (b) SEM image of the CNF mat displaying entangled fibres (scale bar, 5 μm), (c) high-resolution SEM image on individual fibres (scale bar, 200 nm). Random corrugations are visible at the fibre surface. (d) Atomic force microscopic image (height profile) of fibre (scale bar, 500 nm) and corresponding cross-sectional (e) and axial (f) height distributions, respectively. The fibre diameter is ~500 nm and the height of nanocorrugations at the surface varies between 10 and 25 nm. (g) High-resolution TEM image (scale bar, 5 nm) of the edge of the fibre surface and selected area electron diffraction pattern (scale bar, 10 cm) displaying disordered arrangement of crystals. (h) Two important bands in the Raman spectra (that is, D band and G band) appear at 1,363 and 1,586 cm−1. (i) Deconvoluted C1sXPS peak confirms the presence of graphitic carbon and nitrogen atoms in CNFs. Figure 1: Structural and elemental analysis of CNFs. ( a ) Digital image of CNF mat used as catalyst, ( b ) SEM image of the CNF mat displaying entangled fibres (scale bar, 5 μm), ( c ) high-resolution SEM image on individual fibres (scale bar, 200 nm). Random corrugations are visible at the fibre surface. ( d ) Atomic force microscopic image (height profile) of fibre (scale bar, 500 nm) and corresponding cross-sectional ( e ) and axial ( f ) height distributions, respectively. The fibre diameter is ~500 nm and the height of nanocorrugations at the surface varies between 10 and 25 nm. ( g ) High-resolution TEM image (scale bar, 5 nm) of the edge of the fibre surface and selected area electron diffraction pattern (scale bar, 10 cm) displaying disordered arrangement of crystals. ( h ) Two important bands in the Raman spectra (that is, D band and G band) appear at 1,363 and 1,586 cm −1 . ( i ) Deconvoluted C1 s XPS peak confirms the presence of graphitic carbon and nitrogen atoms in CNFs. Full size image In addition to morphological characterizations, the graphitic nature and atomic arrangement was investigated by performing Raman spectroscopy and X-ray photoelectron spectroscopy (XPS). Figure 1h represents the typical Raman spectrum of CNFs indicating two identical peaks that is, D band and G band at ~1,365 and ~1,586 cm −1 , respectively. In general, the G band occurs because of an E 2g hexagonal graphitic lattice, whereas the D band (owing to defects) corresponds to the A 1g mode [23] . In particular, substitution of carbon atoms by other species is accompanied by the introduction of defects into the carbon lattice. The increased D band to G band intensity ratio (I D /I G ), which is nearly one, (~0.81) suggests the presence of defects in the carbon lattice [24] . It is emphasized that nitrogen atoms (as defects) are supposed to be one major component of CNFs. Thus, besides Raman spectroscopy, XPS was also performed to study the atomic configuration of different elements within materials. In the XPS spectrum of CNF, the peaks appearing at binding energy (B.E.) about 400 and 284 eV correspond to the N1 s and C1 s , respectively ( Supplementary Fig. S1 ) [25] . The existence of N1s confirms the presence of nitrogen atoms even if CNFs were pyrolysed at 1,050 °C in Argon media. These results strongly suggest that presence of nitrogen atoms is only due to the native heteroatomic structure of PAN. Further, C1 s peak was fully analysed. The deconvoluted C1 s peak consists of mainly two individual peaks that are assigned to C–C, C=C bond (B.E.~284.8 eV) and C–N bond (B.E.~286.01 eV). An insignificant peak at 287.8 eV was also observed, which indicates the existence of O=C–N type of structures ( Fig. 1i ). CO 2 reduction performance of the CNFs catalyst The CO 2 reduction efficiency of CNFs catalysts has been examined by sweeping the applied voltage from 0.79 to −1.14 V versus the standard hydrogen electrode (SHE) as shown in Fig. 2a . The cyclic voltammetry (CV) curve acquired in the presence of CO 2 −saturated EMIM-BF 4 shows that two well-defined peaks appear at −0.573 V versus SHE and −1.14 V versus SHE, respectively. This first peak is the CO 2 reduction characteristic peak, similar to the results reported (Ag-induced CO 2 reduction) previously [10] , [26] , [27] . To validate the reaction yields at the first peak, the potential was held constant at −0.573 V (versus SHE) and the collected products were analysed by gas chromatography (GC). We observed a Faradaic efficiency of 98% for carbon monoxide (CO) formation. This means that almost all of the energy (electrons) of the system was used for the ‘CO 2 conversion to CO’ process. 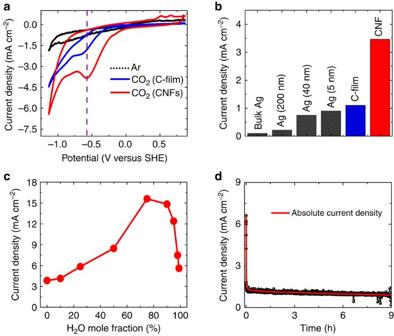Figure 2: Catalytic performance of CNFs for CO2reduction. (a) CVs for CO2reduction in the Ar-saturated (black curve) and CO2-saturated pure EMIM-BF4on carbon film electrode (blue curve) and CNFs electrode (red curve), respectively. The scan rate was 10 mVs−1for both experiments. The vertical pink dashed line represents the potential at which highest CO2reduction in the case of CNF electrode occurs. (b) Absolute current density for CO2reduction at different (bulk Ag, Ag nanoparticles and CNF) electrodes in pure EMIM-BF4electrolyte. CNFs show the highest current density and it is one order of magnitude higher compared with bulk Ag electrode. (c) Current density (at the highest CO2reduction potential) for CNFs catalyst with respect to water mole fraction (%) in EMIM-BF4. (d) Chronoamperogram (absolute current density versus time) for CNFs catalyst at potential 0.573 V versus SHE in pure EMIM-BF4shows the stability of catalyst for the tested duration (9 h). The scan rate was 10 mVs−1. The current densities were obtained based on geometrical surface area. Figure 2: Catalytic performance of CNFs for CO 2 reduction. ( a ) CVs for CO 2 reduction in the Ar-saturated (black curve) and CO 2 -saturated pure EMIM-BF 4 on carbon film electrode (blue curve) and CNFs electrode (red curve), respectively. The scan rate was 10 mVs −1 for both experiments. The vertical pink dashed line represents the potential at which highest CO 2 reduction in the case of CNF electrode occurs. ( b ) Absolute current density for CO 2 reduction at different (bulk Ag, Ag nanoparticles and CNF) electrodes in pure EMIM-BF 4 electrolyte. CNFs show the highest current density and it is one order of magnitude higher compared with bulk Ag electrode. ( c ) Current density (at the highest CO 2 reduction potential) for CNFs catalyst with respect to water mole fraction (%) in EMIM-BF 4 . ( d ) Chronoamperogram (absolute current density versus time) for CNFs catalyst at potential 0.573 V versus SHE in pure EMIM-BF 4 shows the stability of catalyst for the tested duration (9 h). The scan rate was 10 mVs −1 . The current densities were obtained based on geometrical surface area. Full size image To evaluate the role of the corrugated nanofibrillar structure, additional CV experiments were performed with carbon films (C film) prepared by PAN under similar pyrolysis conditions. SEM images clearly demonstrate that C film ( Supplementary Fig. S2 ) neither possesses the overall porosity of nanofibre mats nor the fractal-like corrugations characteristic of the individual fibres. The XPS and Raman spectra analyses ( Supplementary Figs S3–S6 ) confirm a similar chemical structure of C films and CNFs. The first salient feature in the CV curves is that the onset potential for CO 2 reduction (to CO) in CNFs is ~0.23 V lower than that recorded for the C film ( Fig. 2a ). This is indicative of a smaller overpotential for CO 2 reduction in CNFs compared with C film. These results also show that the overpotential in the case of CNFs is similar to that of silver (Ag) catalyst (0.17 V) [4] , the smallest overpotential reported so far. Next, the current density at the highest CO 2 reduction potential for CNFs is approximately two times higher compared with the C film. Figure 2b represents a comparison of the CO 2 reduction (into CO) ability of noble metal Ag film, and Ag nanoparticles (200, 40 and 5 nm) [10] , C film and CNFs electrodes. Ag catalysts are known to be the best catalyst for CO 2 reduction. The comparative analysis delivers remarkably interesting information. The current density for CNFs is ~ 13 times higher than that of the bulk Ag film, 4 times larger than the 5-nm Ag nanoparticles [10] and twice that of the C film-based electrodes (present study). It should be noted that the onset potential is similar but the potential at which maximum CO 2 reduction occurs is significantly lower for CNFs (−0.573 V) in comparison with Ag (for 5 nm Ag nanoparticles, it is −0.75 V) [10] . The potential difference between the maximum CO 2 reduction and hydrogen evolution peak (−1.14 V versus SHE) for the CNF catalyst is larger (0.567 V) compared with Ag nanoparticles (0.45 V) [10] . This opens an adequate potential window for H 2 evolution phenomena, whereas this is not the case using Ag nanoparticles. Utilization of Ag nanoparticles for CO 2 reduction usually results in suppression of H 2 evolution, which is mainly due to the lower potential window between the maximum CO 2 reduction and H 2 evolution peaks. Thus, based on the applied potential, CNFs can be used as a multifunctional catalyst system for both CO formation (−0.573 V versus SHE) and H 2 evolution (−1.14 V versus SHE) and a mixture of CO and H 2 within the applied potential range from −0.573 to −1.14 V versus SHE. This could be an efficient way of producing syngas (CO and H 2 mixture), which can be used directly as fuel (in gas turbines, steam power plants and so on) or as an intermediate for synthesis of higher-energy density fuels (for example, diesel, naphtha and so on). Such features were absent in Ag catalysts. In addition, the electrochemical reduction of CO 2 with respect to proton concentration by varying water mole fraction in electrolyte was also investigated ( Fig. 2c ). The notable advanced reduction current density (approximately five times higher) was observed in EMIM-BF 4 solution (75 mol% water and 25 mol% EMIM-BF 4 ) compared with the pure EMIM-BF 4 . Similar results for Ag nanoparticles have also been reported in our previous work [27] . The addition of water molecules to EMIM-BF 4 instantly influences the pH ( Supplementary Table S1 ) and viscosity of EMIM-BF 4 . The decrease in the pH of the electrolyte solution is caused by the formation of hydroxyl ions (such as [BF 3 OH] − , [BF 2 (OH) 2 ] − and [BF(OH) 3 ] − ) because of hydrolysis of EMIM-BF 4 . This leads to a greater proton availability, which enhances the rate of CO 2 reduction. Moreover, the stability of the catalyst is also one of the major concerns for the development of CO 2 reduction system. Thus, we tested the long-term performance of CNFs catalyst by chronoamperometry (CA) at −0.573 V versus SHE. The current–time CA curve was plotted for the tested duration of 9 h as shown in Fig. 2d . The lower magnitude of tangent (~1.89°, calculated for the curve between 1 and 9 h) proves that the decay in the steady-state current density (in CA curve) is negligible, indicating a higher stability similar to Ag nanoparticles ( Supplementary Fig. S7 ) and demonstrates the renewable characteristics of our catalyst system. It is worth to mention that the initial decrease in the current density (in Fig. 2d ) is due to the mass transport limitation to the electrodes in the absence of stirring or mixing the electrolyte. Once the reactants immediately adjacent to the electrode are consumed, the CO 2 reduction reaction rate is governed by the diffusion of reactant from the bulk to the electrode surface [28] . Thus, a ‘steady-state current density’ is preserved afterwards. Further, a careful evaluation of CV ( Fig. 2a ) and CA ( Fig. 2d ) results illustrates that the current density for CO 2 reduction in CV experiments is more than twice that of the values achieved in CA experiments. It should be noted that the total current measured in CV mode is a combination of Faradaic and charging currents. The charging current arises because of the fluctuation in the double layer capacitance as the applied voltage is changed in CV. However, in a CA experiment (constant potential), the charging current is short lived and decays to a negligible value after several seconds. Thus, the superior current density observed in CV experiments can be attributed to the presence of extra current (due to interface charging) while it is absent in CA experiments [28] . In the next experiment, we measured the work function of CNFs mats and bulk Ag by ultraviolet photoelectron spectroscopy (UPS). Our results indicate that the work function of CNFs (~4.52 eV) is higher than the work function of bulk Ag (4.33 eV). Basically, the binding energies to the catalyst surface are proportional to the average of the electron affinity (work function) of the surface and the electron affinity of the adsorbents. Higher work functions lead to higher binding energies because the energy gained by sharing electrons with the surface is large. Thus, we attribute the high CO 2 reduction performance of CNFs to its unique structural features such as fibrillar morphology, rough surface (due to the fractal-like corrugations on the surface), high number of active catalytic sites and high B.E. of key intermediates to the CNF surface [10] . There are a number of recent reports that explain the low overpotential CO 2 reduction mechanism under various conditions for example, homogenous [11] , [12] or heterogeneous [4] , [10] , [26] system. In particular, Cole et. al [12] suggested that CO 2 conversion in pyridine (liquid) occurs via intermediate pyridinium radical (at negative potential) that further reacts with CO 2 homogeneously to yield products. Rosen et. al [4] , [26] proposed that CO 2 reduction executed in EMIM-BF 4 (electrolyte) occurs through the formation of [EMIM–CO 2 ] intermediate followed by metal catalyst-induced reduction. However, neither of the mechanisms could fully elucidate the CO 2 reduction in the present study because of the heteroatomic nature of our catalyst. The main question, in fact, is how CNFs and intermediate components [EMIM–CO 2 ] take part in CO 2 reduction reaction [26] . There are two electrochemically active species in CNFs catalysts: (i) pyridinic nitrogen and (ii) positively charged carbon atoms. As to counterbalance the high negative charge density on pyridinic N, the adjacent carbon atom carries a substantially higher positive charge density and is an oxidized carbon. If the intriguing CO 2 conversion observed for CNFs is associated to the nitrogen functional groups, the nature of nitrogen atoms should be significantly changed (after the experiment). To examine this, we measured the change in N atom configuration of CNFs catalyst by recording the high-resolution N1 s spectra before and after 9 h electrochemical reaction ( Fig. 3 ). 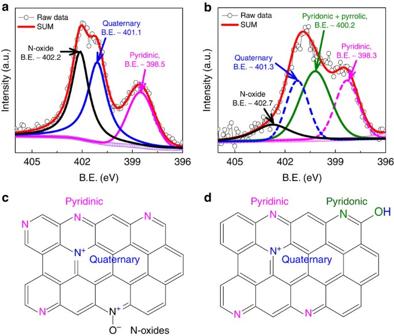Figure 3: Evolution of nitrogen atomic nature in CNFs by XPS. (a) Deconvoluted N1sspectra for CNFs before and (b) after electrochemical experiments. In used catalysts CNFs N1sspectra, N-oxide type of nitrogen content reduced radically and new peak (green solid line) at 400.2 eV (pyridonic N) appears. (c,d) The corresponding atomic structure on the basis of XPS analysis. Figure 3a elucidates the existence of three main nitrogen species that is, pyridinic (B.E.~398.5 eV), quaternary (B.E.~401.1 eV) and nitrogen oxides (B.E.~402.2 eV) in CNFs [29] , [30] . The quantitative analyses demonstrate that the fraction of the various nitrogen species is approximately: 25.8%—pyridinic, 36.7%—quaternary and 37.5%—N-oxide. Interestingly, the N1s spectrum ( Fig. 3b ) acquired for CNFs after 9 h reaction exhibits an additional strong N peak (pyridonic nitrogen) detected at B.E. (~400.1 eV). Our analysis shows that the area of N-oxide peak considerably decreases (37.5–10%) indicating that N-oxides are converted to pyridonic nitrogen (peak area changes from 0 to 37%). However, the electrochemical activity of the CNF catalysts remains unchanged, as proven by CA experiments ( Fig. 2d ), suggesting that N-oxides are not taking part in the CO 2 conversion process. Remarkably, the intensity of the pyridinic (highly active) and quaternary nitrogen (less active) peaks remain approximately constant after the 9 h experiments. If pyridinic nitrogen would directly participate in the reaction, there could be two possible mechanisms. First, pyridinic nitrogen could be permanently protonated, generating quaternary nitrogen [12] resulting in an enhancement in the peak area of quaternary nitrogen, as the B.E. for protonated nitrogen is similar to quaternary (that is, ~401.3 eV) [30] . Alternatively, instead of becoming permanently protonated, pyridinic nitrogens could weakly bind to the CO 2 species in a similar way as in CO 2 reduction by pyridine (homogenous catalyst), resulting in conversion of pyridinic nitrogen into pyridonic species [12] . In both scenarios, a reduction in the peak area of the pyridinic nitrogen peak (after experiments) would have been observed but it remains unchanged (~25.8%) evidencing that such reactions do not take place in our system. These results suggest that direct participation of the nitrogen group in the CO 2 reduction violates the observed renewability of the CO 2 reduction cycle. Thus, N1 s spectra analyses force us to consider that the electrochemical reduction of CO 2 is led by the positively charged carbon atoms. This is further confirmed as nitrogen-free carbon atom catalysts (for example, graphite) exhibit negligible CO 2 reduction current density ( Supplementary Fig. S8 ). The theoretical [18] , [19] and experimental [15] , [31] , [32] studies have also proven that because of high atomic charge and spin density, oxidized carbon atoms can work as effective catalysts for reduction reaction. Initially, the naturally oxidized carbon atoms can be reduced by redox cycling process. At the second step, intermediate complex [EMIM–CO 2 ] will adsorb on reduced carbon atoms and re-oxidize them to their initial state and yield CO as a product ( Fig. 4 ). The cyclic reduction and oxidation process keep the availability of catalytic active carbon atoms for new intermediate complex [EMIM–CO 2 ] adsorption. As a result of the incessant renewable process of active carbon atoms, the CO 2 reduction current density remains almost constant even after 9 h ( Fig. 2d ). This is consistent with a previous report on ORR [15] . Figure 3: Evolution of nitrogen atomic nature in CNFs by XPS. ( a ) Deconvoluted N1 s spectra for CNFs before and ( b ) after electrochemical experiments. In used catalysts CNFs N1 s spectra, N-oxide type of nitrogen content reduced radically and new peak (green solid line) at 400.2 eV (pyridonic N) appears. ( c , d ) The corresponding atomic structure on the basis of XPS analysis. 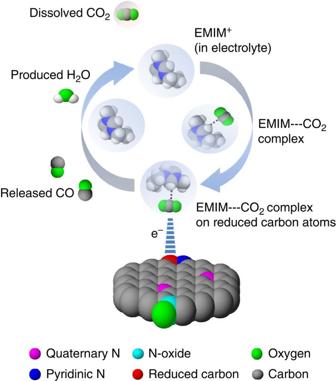Figure 4: CO2reduction mechanism schematic diagram. The CO2reduction reaction takes place in three steps: (1) an intermediate (EMIM–CO2complex) formation, (2) adsorption of EMIM–CO2complex on the reduced carbon atoms and (3) CO formation. Full size image Figure 4: CO 2 reduction mechanism schematic diagram. The CO 2 reduction reaction takes place in three steps: (1) an intermediate (EMIM–CO 2 complex) formation, (2) adsorption of EMIM–CO 2 complex on the reduced carbon atoms and (3) CO formation. Full size image In conclusion, we have uncovered that CNFs, as a metal-free and non-precious catalyst, exhibits exceptionally high current density (~13 times higher than bulk Ag) for a selective conversion of CO 2 to CO (at −0.573 V versus SHE). CNFs can also be potentially used to produce H 2 or a mixture of CO and H 2 (syngas) via tuning the applied potential in the range of −0.573 to −1.14 V versus SHE. The catalytic proficiency of CNFs is attributed to the highly positive charges on carbon atoms due to the existence of the electronegative nitrogen atoms within the carbon lattice. Further, the extremely high CO 2 reduction performance of CNFs catalyst is attributed to the nanofibrillar structure coupled with fractal-like corrugations of the individual fibres, and thus to large extent of active sites. It has also been shown that CNFs exhibits high work function that leads to higher binding energies between the CO 2 intermediate complex and the CNF surface. We propose that non-precious CNFs can successfully replace the expensive noble metal electrodes with the promise of higher performance in the CO 2 conversion. The study also opens up a new avenue for the development of carbon-based heteroatomic catalysts, which can be engineered either by inserting single electronegative components (N, O, S and so on) or a combination of these heteroatoms, for improved CO 2 conversion efficiency. Preparation of CNFs The CNFs were synthesized by electrospinning of polyacrylnitrile (PAN) polymer solution followed by carbonizing the resulted electrospun mat at 1,050 °C in Ar environment [33] , [34] . In brief, a 12-wt% PAN solution was prepared in N , N -dimethylformamide. The nanofibre mat was obtained by electrospinning the PAN solution. During this process, the electric field strength was kept as ~1–2 kV cm −1 . For carbonization, the electrospun nanofibre mat was heated to 350 °C in open air under the heating rate of 7.5 °C min −1 . After it was left at 350 °C for 3 h, the temperature was raised to 1,050 °C at a heating rate of 5 °C min −1 in Ar atmosphere. The sample was kept at 1,050 °C for 1 h and then cooled to room temperature in Ar atmosphere. The nanoscaled fractal-like surfaces of the individual nanofibres form because the carbonization chamber still contains residual oxygen, which partially oxidizes the carbonized surface, whereas the Ar flow blows off loosely connected flakes resulting from this partial surface oxidation. Similar CNFs were used as electrodes in microbial fuel cells and Li-ion batteries, where an enhanced performance was revealed for other electrochemical reactions [34] , [35] , [36] . The C film was also synthesized by carbonizing the film produced from the same solution used to form CNFs followed by similar carbonizing methodology. For C film, the normalized weight with respect to the geometrical surface area was ~16 mg cm −2 , whereas it was ~2.5 mg cm −2 for CNFs sample. The obtained samples were cut in rectangles 1 × 0.5 cm 2 to be used as electrodes for further electrochemical (CO 2 reduction) experiments. Morphological characterization At first, SEM was performed to characterize the morphology of the C film and CNFs. The instrument used for characterization is integrated in a Raith e-LiNE plus ultra-high-resolution electron beam lithography system. During imaging, the samples were kept at a distance of 10 mm from the electron source and the voltage was kept at 10 kV. No particular types of preparation were implemented before imaging. Supplementary Fig. S2 displays the featureless morphology (as expected) of C film compared with CNFs (see Fig. 1b ) synthesized by carbonization of PAN (as precursor). The high-resolution transmission electron microscopy image and selected area electron diffraction pattern of CNFs were acquired by using a JEM-3010 (a 300-kV TEM) with a LaB6 electron source. The TEM was operated at 60 kV accelerating voltage. The samples were prepared by dispersing CNFs fraction in ethanol and the solution was deposited on the holey carbon grid by dripping a dispersion drop. It is emphasized that all the TEM images were captured over the holes in the holey carbon grid, which allowed us to avoid the contrast associated with the carbon film used for support. Images were acquired using a Gatan digital imaging system through Digital Micrograph software. CNFs were also visualized at nanoscale with a Nanoscope IIIa atomic force measurement(atomic force microscopic) digital instrument. First, samples were prepared by dispersing CNFs in methanol followed by drop casting on cleaned Si substrates. The samples were scanned in tapping mode under ambient conditions with a ratio of set point amplitude to the free amplitude of 0.9. Silicon probes Tap190G tips (budget sensor) with typical resonance frequency 190 kHz and radius between 5 and 10 nm were used. Diameters and surface roughness of CNFs were analysed using the section analysis software of the microscope (WSxM 5.0—from Nanotech). Numerous individual CNFs were characterized. The diameter of CNFs varies in the ranges 400–550 nm. Raman spectroscopy Raman spectroscopy (Renishaw Raman 2000) was used to detect the graphitic carbon structure and presence of defects for both CNFs and C film. The spectrum was obtained by exposing small pieces of the samples of CNFs and C film (without any particular treatment) to a 514-nm laser beam (Ar laser, power 10 mW and spot size 10 μm). X-ray photoelectron spectroscopy To execute elemental analysis, XPS experiments were performed using the Kratos Axis-165 instrument. The base pressure of the system was less than 2 × 10 −10 Torr, whereas the pressure during analysis never exceeds 2 × 10 −9 Torr. Samples (before and after electrochemical experiments) were irradiated by a monochromatic Al-K α X-ray source (15 kV, 10 mA). The angle of monochromatic light was fixed at 60° with respect to the sample surface. Photoelectrons were detected by eight channeltrons of the concentric hemispherical analyser over an area of 700 × 300 μm 2 , with a spectrometer take-off angle of zero (with respect to the sample surface normal). The detection was achieved using the constant analyser energy mode. Survey scans were acquired with a pass energy of 160 eV, 1.0 eV step-size and 100 ms dwell time; whereas narrow scans were acquired with a pass energy of 20 eV, 0.1 eV step-size and 200 ms. All scans were performed with the charge-neutralization system running. Charge referencing was done with the adventitious carbon peak position of 284.8 eV. Peak fittings were accomplished using the XPSPEAK version 4.1 program. Baselines were fitted using Shirley-typed backgrounds. All XPS fitting data could be described by a mixture of Gaussian–Lorentzian distributions with typical ratios of 70% Gaussian or higher. Electrochemical experiments To monitor the CO 2 reduction, the following procedure was adapted. Ultra high pure (UHP) Ar (purchased from AirGas) was initially sparged at 1 sl min −1 flow rate and 10 p.s.i. pressure for 2 h until a saturated condition was reached to ensure that all the oxygen was removed from the ionic liquid. CV curve was then taken using a Voltalab PGZ100 potentiostat (purchased from Radiometer Analytical SAS) calibrated with a RCB200 resistor capacitor box. The potentiostat was connected to a personal computer using Volta Master (version 4) software. The obtained curve was used as a reference curve. An aerobic CO 2 (AirGas) was then bubbled in the solution at the same flow rate and pressure for 30 min. The CV curve was then acquired. For better mixing, slight magnetic stirring was applied throughout the entire process. CNFs or C film with 1 × 0.5 cm 2 surface area were used as cathode. The connection between the cathode and the potentiostat was performed using an aluminium crocodile clamp. A 25 × 8-mm 2 piece of platinum, gauze, 52 mesh with 99.9% metal basis (purchased from Sigma-Aldrich) was used as a counter electrode. The reference electrode was a silver wire (0.5 mm diameter, annealed, 99.9% metal basis) purchased from Alfa-Aesar. A solution of ionic liquid EMIM-BF 4 was used as electrolyte (purchased from Sigma-Aldrich). All chemicals were used as purchased without any further chemical treatment. Reference and counter electrodes were washed with acetone and isopropanol several times, rinsed with deionized (DI) water and dried with dry nitrogen (AirGas) before use. The schematic diagram of three-neck electrochemical cell is shown in Supplementary Fig. S9 . The long-term stability of CNFs catalyst was also studied by performing CA experiment at −0.573 V versus SHE in similar electrochemical cell. Additional CV experiments were performed to scan the CO 2 reduction ability of nitrogen-free carbon atom catalysts that is, graphite (see below). Nitrogen-free carbon catalyst performance Graphite chemical structure (hexagonal sp 2 carbon rings) ideally represents the atomic structure of the highly ordered crystallized CNFs. Thus, to do the experiments with nitrogen-free carbon materials, we have chosen graphite as a catalyst. Graphite with >99.9 purity was purchased from the Electron Microscopy Science Company. The cyclic voltammetric (CV) experiments were performed under similar condition (for example, pure ionic liquid—EMIM-BF 4 ) as for CNFs. The typical CV curves obtained in UHP argon and CO 2 -saturated electrolyte are presented in Supplementary Fig. S8 . As expected, both CV curves are fully overlapped to each other, indicating that CO 2 reduction reaction does not take place on the graphite catalyst surface. The observed current density at higher potential can be attributed to the well-studied graphite activity towards hydrogen evolution reaction as reported in previous reports [37] , [38] . These results clearly verify that CO 2 reduction on the nitrogen-free catalyst (graphite) is negligible under the similar experimental conditions. Long-term chronoamperometric study for Ag nanoparticles We also perform the long-term CA experiments for the silver nanoparticles (Ag NPs) to compare the performance with CNFs. The catalyst ink was prepared by mixing 40 mg of Ag NPs purchased from the Aldrich (~40 nm diameter) with 2.4 ml of DI water and 2.4 ml of isopropyl alcohol. To prepare the homogenous dispersion, this mixture was sonicated for 2 min. The electrode was prepared by painting Ag NPs ink onto a piece of Sigracetgraphite layer with 1 cm 2 surface area. The back side of the substrate was fully covered with Hysol 9460 epoxy adhesive. Before measurements, the samples were immersed in 0.1 M sulphuric acid overnight and rinsed with DI water to remove impurities. Electrochemical experiments for Ag NPs were performed in the same condition as for the CNFs samples. As shown in Supplementary Fig. S7 , the magnitude of tangent ~1.84° calculated for the curve between 1 and 9 h is very close to the stability decay slope calculated for CNFs catalysts (~1.89°). Gas chromatography CO formation due to CO 2 reduction was verified by GC in SRI 8610C GC system. The SRI thermal conductivity detector (TCD) consisting of four filaments was set in high current mode. UHP helium (purchased from AirGas) at 10 ml min −1 flow rate was used as a carrier gas. After the TCD detector oven reached 100 °C and stabilized, 2 ml of gas sample was injected to the GC at minute 0.18 and a clear CO peak appeared at minute 3.83. Ultraviolet photoelectron spectroscopy Surface work function measurements were conducted using UPS. The UPS data were acquired with a Physical Electronics PHI 5400 photoelectron spectrometer using He I (21.2 eV) ultraviolet radiation and a pass energy of 8.95 eV. To separate the signal arising from secondary electron emission from the detector from the secondary electron emission from the sample, a −9-V bias was applied to the sample using a battery. How to cite this article: Kumar, B. et al. Renewable and metal-free carbon nanofibre catalysts for carbon dioxide reduction. Nat. Commun. 4:2819 doi: 10.1038/ncomms3819 (2013).